Methylation of allBRCA1copies predicts response to the PARP inhibitor rucaparib in ovarian carcinoma Accurately identifying patients with high-grade serous ovarian carcinoma (HGSOC) who respond to poly(ADP-ribose) polymerase inhibitor (PARPi) therapy is of great clinical importance. Here we show that quantitative BRCA1 methylation analysis provides new insight into PARPi response in preclinical models and ovarian cancer patients. The response of 12 HGSOC patient-derived xenografts (PDX) to the PARPi rucaparib was assessed, with variable dose-dependent responses observed in chemo-naive BRCA1/2 -mutated PDX, and no responses in PDX lacking DNA repair pathway defects. Among BRCA1 -methylated PDX, silencing of all BRCA1 copies predicts rucaparib response, whilst heterozygous methylation is associated with resistance. Analysis of 21 BRCA1- methylated platinum-sensitive recurrent HGSOC (ARIEL2 Part 1 trial) confirmed that homozygous or hemizygous BRCA1 methylation predicts rucaparib clinical response, and that methylation loss can occur after exposure to chemotherapy. Accordingly, quantitative BRCA1 methylation analysis in a pre-treatment biopsy could allow identification of patients most likely to benefit, and facilitate tailoring of PARPi therapy. The development of therapy with poly(ADP-ribose) polymerase inhibitors (PARPi) has been a major advance in the treatment of high-grade serous ovarian carcinoma (HGSOC). PARPi are efficacious in HGSOCs with defective DNA repair by homologous recombination (HR) due to mutation in the breast and ovarian cancer predisposition genes BRCA1 or BRCA2 ( BRCA1/2 ) [1] . When administered as maintenance therapy in the setting of platinum-sensitive relapsed HGSOC, PARPi prolong progression-free survival (PFS), with some patients deriving durable benefit for more than 3 years [2] , [3] , [4] , [5] , [6] . As a result, PARPi are now approved in both the treatment and maintenance settings in relapsed ovarian cancer (OC) by the European Medicines Agency (EMA) and the US Food and Drug Administration (FDA). PARPi may also be relevant as targeted therapy for cancers with a range of defects in HR DNA repair beyond BRCA1/2 mutation. In high-grade OC, HR defects caused by BRCA1/2 mutations are present in 17–25% of cases, of which approximately ¾ are germline and ¼ are somatic [7] , [8] , [9] . Other HR pathway alterations have been documented in an additional 25% of HGSOC [7] , [9] . These HR defects include mutations in the HR pathway genes RAD51C, RAD51D , and PALB2 (6–10%) [7] , [9] , [10] , as well as methylation of BRCA1 (7–17%) [7] , [11] , [12] or RAD51C (1.5–3%) promoters [11] , [13] , which is generally mutually exclusive of BRCA1/2 mutation [7] , [9] , [10] . Despite exciting clinical efficacy, one third of the patients with BRCA1/2 mutant relapsed HGSOC fail to derive benefit from PARPi, with a higher failure rate observed with increasing platinum resistance. Even when patients do respond, the majority relapse within 12 months [3] . A well-defined PARPi resistance mechanism is restoration of HR function via secondary somatic mutations occurring within mutated BRCA1/2 genes, resulting in re-institution of in-frame gene transcription [14] , [15] . Secondary mutations that revert primary BRCA1/2 and RAD51C/D mutations have been described in HGSOC and prostate cancers in association with resistance to both platinum and PARPi therapy [10] , [16] , [17] . Improved understanding of HR defects beyond BRCA1/2 mutations (both primary or secondary) is still required to allow more accurate targeting of PARPi therapy and design of strategies to abrogate PARPi resistance. BRCA1 promoter methylation was first noted 20 years ago in breast cancer [18] , followed by reports in OC [19] , [20] , [21] , [22] . Methylation of CpG sites close to the BRCA1 transcription start site [23] , [24] is associated with reduced BRCA1 mRNA and protein [7] , [13] , [21] , [23] . Accordingly, one of the accepted mechanisms for functional BRCA1 loss involves methylation of one BRCA1 allele combined with a loss of heterozygosity (LOH) event resulting in loss of the other BRCA1 allele [21] . The impact of methylation of a single BRCA1 copy, with retention or demethylation of another, on response to treatment remains unexplored. In support of BRCA1 methylation conferring an HR defect, it has been associated with the same gene expression signature and copy number alterations observed in BRCA1- mutated HGSOC [25] and, more recently, with genomic signatures suggesting HR deficiency in breast cancer [26] . Contrary to these observations, unlike for BRCA1/2 mutations, BRCA1 methylation has not been shown to impact survival in patients with OC, with multiple studies failing to observe a significant improvement in overall survival upon stratification by BRCA1 methylation status [7] , [11] , [27] , [28] . More recently in a clinical trial in triple-negative breast cancer, no benefit was observed for carboplatin in subjects with tumor-associated BRCA1 methylation, compared with BRCA1/2 mutation [29] . Further study of BRCA1 methylation is required to reconcile these observations. Use of PARPi therapy was previously proposed for cancers with BRCA1 methylation [30] . A BRCA1 -methylated breast cancer cell line displayed PARPi sensitivity; and BRCA1 silencing as well as PARPi sensitivity were abolished by the demethylating agent 5-azacytidine [31] . BRCA1 methylation was also weakly associated with response to monotherapy with the PARPi rucaparib in the ARIEL2 Part 1 trial, but it was unclear which BRCA1 -methylated cases would respond to treatment [32] . In contrast, in a study of long-term responders following maintenance therapy with PARPi after response to platinum, no long-term responders (>2 years) were found to have BRCA1 methylation in their archival HGSOC [33] . Thus, the likelihood of PARPi response in patients with BRCA1- methylated HGSOC requires clarification. Variable levels of BRCA1 promoter methylation, ranging from 5 to 100%, have been previously reported in breast and OC samples, with most studies assigning “methylation” status to samples when as little as 5–15% methylation is detected [13] , [25] , [27] , [33] . In some cases, this is consistent with low neoplastic cellularity. However, the possibility that methylation of all BRCA1 copies might be required to impact therapeutic outcome has not yet been addressed. Here we test the hypothesis that the zygosity status of BRCA1 methylation (homozygous or hemizygous vs. heterozygous) may have an impact on PARPi or platinum response and may be affected by treatment pressure, allowing for the rapid development of drug resistance. The terms “homozygous” and “homozygosity” used to define the methylation status in this paper will cover all cases where unmethylated alleles are absent, regardless of the BRCA1 copy number (Supplementary Fig. 1 ). Here we show that the rucaparib response of BRCA1 -methylated OC cell lines and patient-derived xenografts (PDX) depends upon the BRCA1 methylation zygosity. Further, we report quantitative methylation analysis of pre-treatment HGSOC samples from the ARIEL2 Part 1 PARPi trial, which is the only published clinical trial to date for which pre-treatment biopsies of cases documented to contain BRCA1 methylation are available. In this clinical trial setting, we also demonstrate that BRCA1 methylation zygosity correlates with rucaparib response. Genomic characterization of HGSOC PDX For this study, we have characterized PDX from 12 HGSOC patients, ten who were chemotherapy naive and two who had received multiple prior lines of therapy. Histologic assessment and WT1, PAX8, and p53 immunohistochemistry (IHC) staining confirmed that the PDX retained HGSOC features that were observed in the baseline carcinoma (Fig. 1a , Supplementary Fig. 2 ) [34] . The patient HGSOC and/or PDX whole tumor DNA samples were profiled using the Foundation Medicine T5a next-generation sequencing (NGS)-based test and RNA sequencing (RNA-seq). In addition, each PDX was also capture-sequenced for mutations in DNA repair pathway genes, in particular mutations that could cause HR deficiency, as previously described [9] , and tested for BRCA1 promoter methylation. Apart from the expected somatic mutations in TP53 [35] , mutations were also identified in BRCA1/2 in four HGSOC, one of which was confirmed to be germline (#56; Fig. 1b , Supplementary Fig. 3a , Supplementary Data 1 ). Other events that are commonly detected in HGSOC included RB1 mutation or deletion in six cases (#56, 19, 11, 169, 27, 80), NF1 deletion in one case (#80), and CCNE1 amplification in two cases (#29, 201). RNA-seq analysis, performed on the baseline patient HGSOC samples used to generate the PDX, confirmed the reduced expression of deleted genes and high expression of amplified genes (Fig. 1c , Supplementary Fig. 3b ). In addition to deleterious BRCA1/2 mutations in four HGSOC, BRCA1 methylation was detected in four of the 12 HGSOC and in the corresponding PDX (#11, 62, 48, 169) [34] . The remaining four PDX were assigned an HR-DNA repair gene wild-type status, since no pathogenic mutations were detected in a curated set of HR pathway genes (Fig. 1b ). Fig. 1 Genomic profiling of 12 HGSOC PDX. a IHC staining of PAX8, WT1, and p53 of passage one (T1) PDX tumors. Loss of p53 expression was observed for PDX #54 with a frameshift TP53 mutation (p.G199fs*8), #11 with a nonsense TP53 mutation (p.E198*), and #80 with a splice site TP53 mutation (IVS6-1G>T). b Select genomic events detected by the Foundation Medicine T5a test, BROCA assay, and BRCA1 promoter methylation testing. The Foundation Medicine T5a test was performed on PDX samples, except for case #48, where it was performed on patient HGSOC material. T5a test results and BROCA v4 assay results for PDX #11, #13, #27, #29, #56, and #62 were previously published [34] ; BROCA v6 was performed for all other PDX [34] . c RNA-seq gene expression for genes with detected mutations or copy number changes. RNA-seq was performed on baseline patient HGSOC material samples. RNA-seq was also performed on PDX #169 and #201 samples, to verify expression levels observed in the matched HGSOC with suboptimal sample quality due to either low neoplastic cellularity or poor RNA quality (#80 inadequate quality); rep—RNA-seq library replicate Full size image Dose-dependent rucaparib responses in BRCA1/2 mutant PDX To assess PARPi sensitivity, rucaparib was delivered by oral gavage 5 days a week for 3 weeks at one of the three dose levels—150, 300, or 450 mg kg −1 . 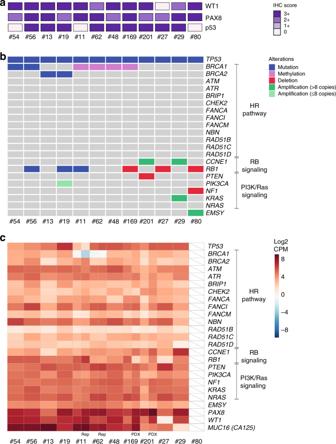Fig. 1 Genomic profiling of 12 HGSOC PDX.aIHC staining of PAX8, WT1, and p53 of passage one (T1) PDX tumors. Loss of p53 expression was observed for PDX #54 with a frameshiftTP53mutation (p.G199fs*8), #11 with a nonsenseTP53mutation (p.E198*), and #80 with a splice siteTP53mutation (IVS6-1G>T).bSelect genomic events detected by the Foundation Medicine T5a test, BROCA assay, andBRCA1promoter methylation testing. The Foundation Medicine T5a test was performed on PDX samples, except for case #48, where it was performed on patient HGSOC material. T5a test results and BROCA v4 assay results for PDX #11, #13, #27, #29, #56, and #62 were previously published34; BROCA v6 was performed for all other PDX34.cRNA-seq gene expression for genes with detected mutations or copy number changes. RNA-seq was performed on baseline patient HGSOC material samples. RNA-seq was also performed on PDX #169 and #201 samples, to verify expression levels observed in the matched HGSOC with suboptimal sample quality due to either low neoplastic cellularity or poor RNA quality (#80 inadequate quality); rep—RNA-seq library replicate As expected, three of four PDX that were HR deficient due to BRCA1/2 mutations responded to rucaparib in vivo (Table 1 , Supplementary Data 2 ). Some mice bearing PDX #19 or #56 obtained durable regressions lasting more than 80 days (Fig. 2a, b ). Despite being tested in the chemo-naive/first-line setting, without prior exposure to chemotherapy or PARPi, variable dose-dependent responses were observed, and not all BRCA1/2 mutant HGSOC PDX were equally sensitive to PARPi (Table 1 , Fig. 2a, b , Supplementary Fig. 4a, b ). Table 1 Responses observed in 12 HGSOC PDX to cisplatin and rucaparib treatment in vivo Full size table Fig. 2 Cisplatin and rucaparib responses in BRCA1/2 mutant and HR wild-type HGSOC PDX. Rucaparib and cisplatin response in a PDX #56 ( BRCA1 mutant); b PDX #19 ( BRCA2 mutant); c PDX #201 (HR-DNA repair gene wild-type); and d PDX #29 (HR-DNA repair gene wild-type). Recipient mice bearing PDX were randomized to treatment with vehicle or rucaparib, at the dose shown. PDX were harvested at a tumor volume of 600–700 mm 3 . Cisplatin response data for PDX #19, #56, and #29 were previously published [34] . See Table 1 and Supplementary Data 2 for median TTH and p -values for survival comparison. Mean tumor volume (mm 3 ) ± 95% CI (hashed lines are representing individual mice) and corresponding Kaplan–Meier survival analysis. Censored events are represented by crosses on Kaplan–Meier plot; n = individual mice Full size image Two of four BRCA1/2 mutant PDX responded to the lowest dose of rucaparib tested: BRCA2 mutant PDX #19 (median time to harvest (TTH) 74 days vs. vehicle 22 days, p = 0.012, log-rank test, n = 4, 21) and BRCA1 mutant PDX #56 (median TTH 67 days vs. vehicle 15 days, p = 0.003, log-rank test, n = 5, 16) at 150 mg kg −1 . The chemo-naive BRCA2 mutant PDX #13 had a statistically significant response to both 300 and 450 mg kg −1 rucaparib, with median TTH of 81 days for rucaparib 300 mg kg −1 vs. 43 days for vehicle ( p = 0.01, log-rank test, n = 9, 22), although regressions were not observed. Strikingly, PDX #54, with a pathogenic missense BRCA1 BRCT domain mutation (c.5095C>T, p.R1699W), was refractory to rucaparib in the first-line setting (median TTH for rucaparib 300 mg kg −1 36 days vs. vehicle 32 days, p = 0.9, log-rank test, n = 9, 4), possibly due to HSP90-mediated stabilization of the mutant BRCA1 protein, as has been observed with other BRCT domain-mutant BRCA1 proteins [36] . In further experiments, DNA sequencing failed to detect any secondary mutations in either BRCA1 or BRCA2 in these four PDX at recurrence (Supplementary Data 3 ). Variable rucaparib responses in PDX with BRCA1 methylation In keeping with the proposed requirement of an HR defect for PARPi response, the four PDX derived from HGSOC lacking mutation of HR genes and BRCA1 promoter methylation showed no evidence of tumor regression or disease stabilization with rucaparib (Table 1 , Fig. 2c, d , Supplementary Fig. 4c, d ). In contrast, variable rucaparib responses were observed in models with BRCA1 methylation. Two chemo-naive baseline patient HGSOC samples and the corresponding PDX (#11 and #62), in which no pathogenic HR gene mutations were detected, were found to harbor BRCA1 methylation by methylation-specific PCR (MSP) as previously reported (Fig. 1b ) [34] . Furthermore, two baseline patient HGSOC samples obtained from patients who had received prior treatment in the clinic and their corresponding PDX (#48 and #169) were also found to harbor BRCA1 methylation by MSP. No other pathogenic events in HR pathway genes were identified in these four HGSOC or corresponding PDX (Fig. 1b ). The methylation status of these PDX samples was re-assessed by both methylation-specific high-resolution melting (MS-HRM) and methylation-sensitive droplet digital PCR (MS-ddPCR). Seven co-methylated CpG sites of the BRCA1 promoter region were assessed; MS-HRM (−37, −29, −21, and −19) [37] and ddPCR (+14, +16, and +19). Two modes of BRCA1 methylation were observed, with (i) homozygous methylation on all BRCA1 copies present and (ii) heterozygous methylation where both methylated and unmethylated copies were observed (Fig. 3a, b , Supplementary Figs. 1 and 5 ). The two chemo-naive PDX (#11 and #62) were consistently found to harbor ~100% BRCA1 methylation and hence were assigned a homozygous status. The two PDX from HGSOC from patients treated with multiple lines of prior therapy (#48 and #169) were consistently found to harbor around 50% methylation and, therefore, were assigned a heterozygous status. The presence of two peaks in the MS-HRM analysis indicated that methylation was concordant across the four sites, as molecules with partial methylation would have intermediate melting temperatures and form more complex patterns (Supplementary Fig. 5 ). Analysis of the matched source patient HGSOC samples was also consistent with homozygous (#11 and #62) and heterozygous (#48 and #169) methylation of the BRCA1 promoter, although due to variable neoplastic purity in patient HGSOC samples, it was more challenging to estimate the proportion of methylated copies (Supplementary Data 4 ). RNA-seq, BRCA1 quantitative reverse transcription PCR (qRT-PCR) and western blotting (WB) analysis showed markedly reduced BRCA1 expression in the two source patient HGSOC samples and matched PDX models with homozygous methylation, but not in the two with heterozygous methylation, further supporting that methylation, mutation, or loss of all copies is required for BRCA1 silencing (Supplementary Fig. 6a–c , Supplementary Table 1 ) [26] . We assessed HR pathway activity by ex vivo RAD51 foci formation assay, which showed formation of RAD51 foci in response to DNA damage in PDX #169, which harbored heterozygous methylation, but not in PDX #11 or PDX #62, which both harbored homozygous methylation (Fig. 3c, d , Supplementary Fig. 7 ). Fig. 3 BRCA1 promoter methylation in HGSOC PDX and rucaparib response. a A diagram of two modes of BRCA1 promoter methylation observed in four PDX #11, #62, #48, and #169. Homozygous methylation status was assigned when % of methylation was close to 100%, therefore all observed copies were methylated. Heterozygous methylation status was assigned when both, methylated and unmethylated, copies were observed. b BRCA1 methylation in four HGSOC PDX (#62, #48, #169, #11) assessed by MS-ddPCR (mean ± 95% CI); n = 2–3 mice for each treatment and PDX model. c RAD51 foci formation 4 h after 10 Gy irradiation was observed in PDX #169 with heterozygous BRCA1 methylation and not in PDX #11 and PDX #62 with homozygous BRCA1 methylation. d Quantification of ex vivo γH2AX and RAD51 foci formation in geminin-positive cells 4 h after 10 Gy irradiation (mean ± 95% CI). γH2AX foci are observed at the sites of DNA damage, and RAD51 foci are observed at the sites of HR pathway repair; n = 12 (four fields of view from three independent experiments) for each treatment and PDX model. Untreated and irradiated cells were compared by multiple t -tests for γH2AX and RAD51 foci formation. *** p < 0.001; ns not significant. e Responses to cisplatin and rucaparib in vivo treatment observed in chemo-naive PDX #62 with homozygous BRCA1 methylation. f RECIST 1.1 measurements of three monitored tumor lesions in patient #11, with homozygous methylation of BRCA1 , treated with rucaparib. g CT scans of the two largest monitored lesions prior to and during rucaparib treatment of the patient #11. h , i Responses to cisplatin and rucaparib in vivo treatment observed in PDX #48 and #169 with heterozygous BRCA1 methylation. Recipient mice bearing PDX were randomized to treatment with vehicle or rucaparib, at the dose shown. PDX were harvested at a tumor volume of 600–700 mm 3 (see Table 1 and Supplementary Data 2 for median TTH and p -values for survival comparison). Mean tumor volume (mm 3 ) ± 95% CI (hashed lines are representing individual mice) and corresponding Kaplan–Meier survival analysis. Censored events are represented by crosses on Kaplan–Meier plot; n = individual mice. HOM homozygous, HET heterozygous Full size image One of the two chemo-naive PDX with homozygous BRCA1 promoter methylation (#62) responded to 300 mg kg −1 rucaparib, with tumor regressions observed in two of seven mice (median TTH 71 days vs. vehicle 18 days, p < 0.001, log-rank test, n = 7, 11) (Table 1 , Fig. 3e ). This was notable, given that PDX #62 was resistant/refractory to cisplatin (defined as three or more mice with tumor progressing during cisplatin treatment) and was characterized by the presence of multiple oncogene amplifications (Table 1 ) [34] . The other PDX with homozygous BRCA1 methylation (#11), despite being exquisitely sensitive to platinum [34] , failed to respond to rucaparib at the low dose tested (150 mg kg −1 ) but was not exposed to 300 and 450 mg kg −1 (Supplementary Data 2 , Supplementary Fig. 6d ). However, the patient from whom PDX #11 was derived subsequently received single-agent rucaparib with starting dose of 600 mg twice daily and had a partial response (PR) of 10 months as demonstrated by Response Evaluation Criteria In Solid Tumors version 1.1 (RECIST 1.1) (Fig. 3f, g ), suggesting that in the PDX, a higher dose of rucaparib treatment in vivo may have been efficacious. Conversely, no disease stabilization or tumor regression was observed in response to rucaparib for either PDX #48 or #169 both of which harbored heterozygous BRCA1 promoter methylation (Table 1 , Fig. 3h, i ). In terms of the corresponding patient courses, case #48 progressed 4 months following third-line platinum therapy, at which point the disease was biopsied (PDX established) and she was subsequently treated with single-agent PARPi therapy, progressing after just 2 months. Case #169 had platinum refractory disease and progressed within 1 month of first-line carboplatin/paclitaxel chemotherapy (PDX established from ascites) and did not receive a PARPi. Importantly, the heterozygous BRCA1 methylation status in both cases reflected a change from baseline. DNA from archival patient HGSOC samples for cases #48 and #169 revealed homozygous BRCA1 methylation in chemotherapy-naive ascites collected at diagnosis for both cases and also in the surgical debulking samples following neoadjuvant chemotherapy for both cases (Supplementary Data 4 ). BRCA1 promoter methylation was also examined in PDX samples upon cancer recurrence following in vivo treatment with either cisplatin or rucaparib. No loss of homozygous BRCA1 methylation was observed for either PDX #11 or #62 following treatment with rucaparib or cisplatin (Fig. 3b ). Similarly, no loss of heterozygous BRCA1 methylation or gain of homozygous methylation was observed for either PDX #48 or #169 following treatment with either cisplatin or rucaparib (Fig. 3b ). Variable rucaparib responses in BRCA1 -methylated cell lines To further study whether BRCA1 promoter methylation predisposes OC cells to rucaparib response through loss of the HR pathway activity, we generated a cell line from PDX #62 (WEHICS62) that retained homozygous BRCA1 methylation. Reduced expression of BRCA1 mRNA, consistent with silencing of BRCA1 , was observed in RNA-seq and qRT-PCR analysis of the WEHICS62 cell line (two samples), the matched PDX (six samples), and the baseline patient HGSOC sample, compared to a PDX with unmethylated wild-type BRCA1 (Supplementary Fig. 6b , Supplementary Fig. 8 ). 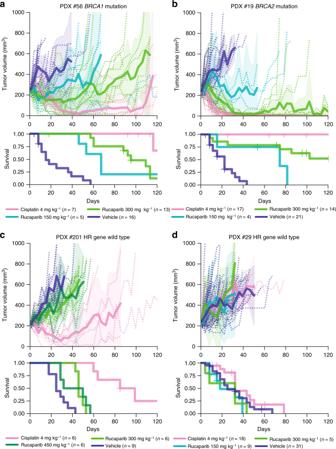Fig. 2 Cisplatin and rucaparib responses inBRCA1/2mutant and HR wild-type HGSOC PDX. Rucaparib and cisplatin response inaPDX #56 (BRCA1mutant);bPDX #19 (BRCA2mutant);cPDX #201 (HR-DNA repair gene wild-type); anddPDX #29 (HR-DNA repair gene wild-type). Recipient mice bearing PDX were randomized to treatment with vehicle or rucaparib, at the dose shown. PDX were harvested at a tumor volume of 600–700 mm3. Cisplatin response data for PDX #19, #56, and #29 were previously published34. See Table1and Supplementary Data2for median TTH andp-values for survival comparison. Mean tumor volume (mm3) ± 95% CI (hashed lines are representing individual mice) and corresponding Kaplan–Meier survival analysis. Censored events are represented by crosses on Kaplan–Meier plot;n= individual mice In contrast, OVCAR8, a cell line generated from a patient with OC refractory to carboplatin [38] , [39] and previously reported to harbor BRCA1 methylation [40] , was found to have heterozygous BRCA1 methylation when assessed by quantitative MS-ddPCR (~66% methylation with three copies of BRCA1 , likely two methylated copies and one unmethylated copy) (Supplementary Table 2 – 3 , Supplementary Fig. 9 ). Furthermore, BRCA1 expression was detected by qRT-PCR (Supplementary Fig. 6b ). This finding was in keeping with our previous report of the ability of OVCAR8 cells to form RAD51 foci and resistance of the OVCAR8 cell line to both platinum and PARPi agents in vitro, both consistent with a competent HR pathway [17] . The homozygous BRCA1 -methylated cell line, WEHICS62, had a reduced capacity to form RAD51 foci in response to IR damage, as did an HR-deficient cell line derivative of OVCAR8 (with RAD51C KO), when compared to the heterozygous BRCA1 -methylated OVCAR8 cell line, a second HR-competent OC cell line, OV90, or a normal immortalized fallopian tube epithelial cell line, FT282 [41] (Fig. 4a, b ). Colony formation and cell proliferation analyses revealed that WEHICS62 cells were sensitive to rucaparib, as were the HR-deficient cell line derivative of OVCAR8 (with RAD51C KO) and the BRCA2 -mutant OC cell line PEO1 [42] . In comparison, the parental OVCAR8 cell line with heterozygous BRCA1 promoter methylation and the HR-competent PEO4 OC cell line were not sensitive to rucaparib in vitro (Fig. 4c, d ). Fig. 4 Assessment of HR deficiency and rucaparib sensitivity in BRCA1 -methylated cell lines. a RAD51 foci formation assessed 6 h post exposure to 10 Gy irradiation in HR-competent OC cell line (OV90), immortalized fallopian tube cell line (FT282), OC cell line with heterozygous BRCA1 methylation (OVCAR8), OVCAR8 derivative with RAD51C KO, and HGSOC cell line with homozygous BRCA1 methylation (WEHICS62). b Quantification of RAD51 foci formation in EdU-positive cells for OV90, FT282, OVCAR8, OVCAR8 derivative with RAD51C KO, and WEHICS62. RAD51 foci formation ability was compared to the untreated controls. At least 170 EdU-positive cells were counted for each cell type and treatment (multiple fields of view from three independent experiments). Mean ± SEM. c Colony formation assay assessing rucaparib response at 14 days in HR-competent OC cell line (PEO4), at 10 days in OC cell line with heterozygous BRCA1 methylation (OVCAR8) and HR-deficient OC cell line (PEO1), and at 21 days in HGSOC cell line with homozygous BRCA1 methylation (WEHICS62); n = 3 independent experiments. Mean ± SEM. d In vitro rucaparib response assessed by cell count proliferation time course assay using IncuCyte ZOOM of OC cell lines OVCAR8, OVCAR8 derivative with RAD51C KO and WEHICS62. One of three similar independent experiments shown. Mean ± SEM; * denotes p < 0.05 for post-IR WEHICS62 % comparison with irradiated OVCAR8 and OV90 counterparts. IR irradiated, Cntrl untreated control, ND not detected Full size image Rucaparib response in patients with BRCA1 -methylated HGSOC To investigate whether heterozygous and homozygous BRCA1 promoter methylation correlated with PARPi response in clinical samples, we used quantitative MS-ddPCR to analyze the archival and pre-treatment (study-entry) tumor biopsies from 21 patients who were identified to have BRCA1 -methylated HGSOC from the cohort of 204 patients treated on the ARIEL2 Part 1 single-agent rucaparib trial [32] (detail provided in methods, Table 2 , Supplementary Data 5 ). To determine BRCA1 methylation percentage and zygosity status in tumor cells, the raw MS-ddPCR percentage of methylated copies was adjusted for neoplastic cellularity and BRCA1 copy number. This adjustment was required because the expected proportion of observed unmethylated copies is dependent on the ratio of unmethylated somatic copies to tumor copies at the BRCA1 locus. 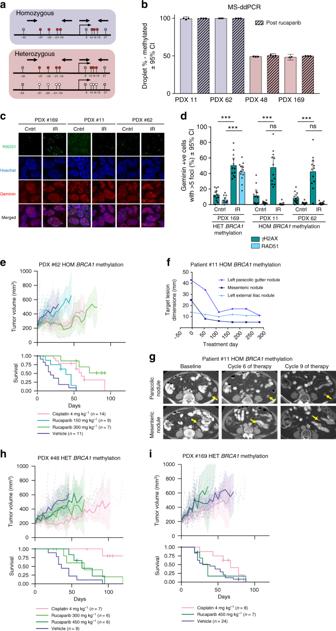Fig. 3 BRCA1promoter methylation in HGSOC PDX and rucaparib response.aA diagram of two modes ofBRCA1promoter methylation observed in four PDX #11, #62, #48, and #169. Homozygous methylation status was assigned when % of methylation was close to 100%, therefore all observed copies were methylated. Heterozygous methylation status was assigned when both, methylated and unmethylated, copies were observed.bBRCA1methylation in four HGSOC PDX (#62, #48, #169, #11) assessed by MS-ddPCR (mean ± 95% CI);n= 2–3 mice for each treatment and PDX model.cRAD51 foci formation 4 h after 10 Gy irradiation was observed in PDX #169 with heterozygousBRCA1methylation and not in PDX #11 and PDX #62 with homozygousBRCA1methylation.dQuantification of ex vivo γH2AX and RAD51 foci formation in geminin-positive cells 4 h after 10 Gy irradiation (mean ± 95% CI). γH2AX foci are observed at the sites of DNA damage, and RAD51 foci are observed at the sites of HR pathway repair;n= 12 (four fields of view from three independent experiments) for each treatment and PDX model. Untreated and irradiated cells were compared by multiplet-tests for γH2AX and RAD51 foci formation. ***p< 0.001; ns not significant.eResponses to cisplatin and rucaparib in vivo treatment observed in chemo-naive PDX #62 with homozygousBRCA1methylation.fRECIST 1.1 measurements of three monitored tumor lesions in patient #11, with homozygous methylation ofBRCA1, treated with rucaparib.gCT scans of the two largest monitored lesions prior to and during rucaparib treatment of the patient #11.h,iResponses to cisplatin and rucaparib in vivo treatment observed in PDX #48 and #169 with heterozygousBRCA1methylation. Recipient mice bearing PDX were randomized to treatment with vehicle or rucaparib, at the dose shown. PDX were harvested at a tumor volume of 600–700 mm3(see Table1and Supplementary Data2for median TTH andp-values for survival comparison). Mean tumor volume (mm3) ± 95% CI (hashed lines are representing individual mice) and corresponding Kaplan–Meier survival analysis. Censored events are represented by crosses on Kaplan–Meier plot;n= individual mice. HOM homozygous, HET heterozygous A BRCA1 copy number of 1 was assigned in cases where LOH was consistently predicted by both the Foundation Medicine T5 test and the BROCA assay and a copy number of 1 was reported by the Foundation Medicine T5 test. Cases that had a single methylated BRCA1 locus and deletion of the second allele were classified as homozygous for BRCA1 methylation. Low estimated neoplastic cellularity (of 20%) precluded accurate determination of BRCA1 methylation zygosity in five out of 32 samples (archival and/or pre-treatment) tested from the 21 cases. Archival BRCA1 methylation zygosity status could be determined with high confidence for 17 cases: ten cases were homozygous and seven cases were heterozygous (four of which had surgery at the time of diagnosis). Table 2 Degree of BRCA1 methylation in HGSOC where a pre-treatment biopsy was available for analysis in the ARIEL2 Part 1 clinical trial Full size table In order to assess the impact of BRCA1 methylation zygosity on PARPi response, as determined at the time of treatment commencement, we focused on ARIEL2 cases for which pre-treatment biopsy samples were available for BRCA1 methylation analysis. For 12 of the 21 BRCA1 -methylated cases, sufficient material from pre-treatment tumor biopsies was available (Supplementary Data 5 ). Eight of the 12 cases (#15–21) had homozygous BRCA1 methylation in the pre-treatment tumor biopsy, six of these (#16–21) were high confidence calls based on neoplastic cellularity of >20% (these six cases are hereafter referred to as the homozygous BRCA1 methylation (high confidence) subgroup). Two of the 12 cases with material available for analysis (#1, 2) had homozygous and heterozygous BRCA1 methylation, respectively, in the archival sample, and no evidence of methylation in the pre-treatment tumor biopsy (Table 2 ), consistent with loss of methylation. Two final cases (#7, 8) had heterozygous BRCA1 methylation in both the archival sample and matched pre-treatment tumor biopsy. We hypothesized that patients with homozygous BRCA1 methylation (high confidence) at the time of enrollment into the trial ( n = 6) would respond similarly to the BRCA1/2 mutant subgroup with higher response rates and a longer PFS than patients with BRCA1/2 wild-type tumors that had never been observed to have any BRCA1 methylation ( BRCA1/2 wild-type non- BRCA1 -methylated). The homozygous BRCA1 methylation (high confidence) subgroup had a median PFS of 14.5 months (95% CI 4.8–18.3, n = 6) comparable to the BRCA1/2 mutant subgroup (12.8 months, 95% CI 9.0–14.7, n = 40). Whilst not statistically significant, the PFS was longer for the high-confidence homozygous BRCA1 -methylated group when compared to BRCA1/2 wild-type non- BRCA1 -methylated cases (5.5 months, 95% CI 5.0–6.2, p = 0.062, log-rank test, n = 143) (Fig. 5a ). Fig. 5 Homozygous BRCA1 methylation and rucaparib response in the ARIEL2 Part 1 trial. a Kaplan–Meier progression-free survival analysis of patients with HGSOC with homozygous BRCA1 methylation in the pre-treatment tumor biopsy, which was of high confidence based on adequate neoplastic cellularity (homozygous BRCA1 methylation (high confidence)), compared with patients with HGSOC in which there had ever been any other evidence of BRCA1 methylation (ever any BRCA1 methylation), compared with all other patients in the ARIEL2 Part 1 trial without any BRCA1 methylation ( BRCA1/2 mutant vs. BRCA1/2 wild-type non- BRCA1 -methylated subgroups). Shaded areas represent 95% CI for homozygous BRCA1 methylation (high confidence) and ever any BRCA1 methylation, other groups. b Genome-wide LOH % assessed in the pre-treatment biopsies compared across subgroups: homozygous BRCA1 methylation (high-confidence), ( n = 6); ever any BRCA1 methylation, ( n = 6); BRCA1/2 mutant, ( n = 27); and BRCA1/2 wild-type non- BRCA1 -methylated, ( n = 96). Boxplot—median, whiskers—95% CI, dots represent individual samples. c Best percentage change from baseline in sum of longest diameter of target lesions according to RECIST 1.1 compared across subgroups: homozygous BRCA1 methylation (high confidence), ( n = 6); ever any BRCA1 methylation, ( n = 15); BRCA1/2 mutant, ( n = 40); and BRCA1/2 wild-type non- BRCA1 -methylated, ( n = 143). Boxplot—median, whiskers—95% CI, dots represent individual samples. d Best percentage change from baseline in sum of longest diameter of target lesions according to RECIST 1.1 in the BRCA wild-type LOH-high subgroup of patients by BRCA1 methylation status. Each bar represents percentage change from baseline in sum of the longest diameter of target lesions for an individual patient according to RECIST 1.1. In some patients, although best percentage change of >30% was observed, the response was not investigator confirmed and thus classified as stable disease (SD) or progressive disease (PD). PR partial response, PD progressive disease, SD stable disease, CR complete response Full size image All homozygous BRCA1 methylation samples had high genomic LOH scores (>16%), an indirect marker of potential HR deficiency through genomic scarring [6] (Fig. 5b , Supplementary Fig. 10a ). The mean LOH score for homozygous BRCA1 -methylated cases was significantly higher than for BRCA1/2 wild-type non- BRCA1 -methylated cases (27.9 vs. 15.9, p = 0.04, independent t -test). There were no significant differences observed in the mean genomic LOH scores between the homozygous BRCA1 methylation subgroup and the subgroup of other cases which had ever had any BRCA1 methylation (Table 2 , Fig. 5b , Supplementary Fig. 10a ), indicating that these samples may have harbored homozygous BRCA1 methylation in the past, leading to accumulation of genomic scarring. 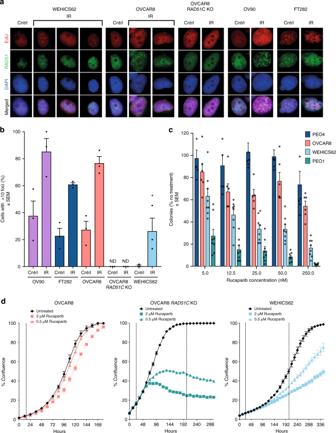Fig. 4 Assessment of HR deficiency and rucaparib sensitivity inBRCA1-methylated cell lines.aRAD51 foci formation assessed 6 h post exposure to 10 Gy irradiation in HR-competent OC cell line (OV90), immortalized fallopian tube cell line (FT282), OC cell line with heterozygousBRCA1methylation (OVCAR8), OVCAR8 derivative withRAD51CKO, and HGSOC cell line with homozygousBRCA1methylation (WEHICS62).bQuantification of RAD51 foci formation in EdU-positive cells for OV90, FT282, OVCAR8, OVCAR8 derivative withRAD51CKO, and WEHICS62. RAD51 foci formation ability was compared to the untreated controls. At least 170 EdU-positive cells were counted for each cell type and treatment (multiple fields of view from three independent experiments). Mean ± SEM.cColony formation assay assessing rucaparib response at 14 days in HR-competent OC cell line (PEO4), at 10 days in OC cell line with heterozygousBRCA1methylation (OVCAR8) and HR-deficient OC cell line (PEO1), and at 21 days in HGSOC cell line with homozygousBRCA1methylation (WEHICS62);n= 3 independent experiments. Mean ± SEM.dIn vitro rucaparib response assessed by cell count proliferation time course assay using IncuCyte ZOOM of OC cell lines OVCAR8, OVCAR8 derivative withRAD51CKO and WEHICS62. One of three similar independent experiments shown. Mean ± SEM; * denotesp< 0.05 for post-IR WEHICS62 % comparison with irradiated OVCAR8 and OV90 counterparts. IR irradiated, Cntrl untreated control, ND not detected The objective response rates in the high confidence homozygous BRCA1 -methylated subgroup were significantly better compared to BRCA1/2 wild-type non- BRCA1 -methylated cases ( n = 143 cases, p = 0.0014, Fisher Exact test, Supplementary Table 4 ), with five of six (83%) patients with homozygous BRCA1 methylation detected in the pre-treatment biopsy achieving a PR and the sixth patient having a 33% reduction in target lesions that was not confirmed by subsequent CT scanning and was classified instead as stable disease (SD). A significant difference in reduction in the mean change in target lesion sizes was observed between the homozygous BRCA1 -methylated groups and BRCA1/2 wild-type non- BRCA1 -methylated cases (−53.9 vs. −13.5%, p = 0.001, independent t -test, Fig. 5c, d , Supplementary Fig. 10b ). These findings indicated that cases with confirmed homozygous BRCA1 promoter methylation were more likely to respond to rucaparib. To improve our understanding of the sensitivity and resistance mechanisms to PARP inhibitors, both primary and acquired, we assessed the in vivo rucaparib response of 12 chemo-naive or post-treatment HGSOC PDX. Variable responses to rucaparib were observed in the four chemo-naive HGSOC PDX with BRCA1/2 mutations, ranging from complete response (CR) to progressive disease. Of note, PARPi response has not been tested in the chemo-naive setting in the clinic, but our results were in keeping with the range of single-agent PARPi responses reported for patients with recurrent BRCA1/2 mutant HGSOC [1] , [32] , [43] . We also explored mechanisms of acquired PARPi resistance by screening post-rucaparib treated PDX samples for the presence of reversion or secondary BRCA1/2 mutations and none were observed. None of the four PDX thought to be HR proficient showed regression or disease stabilization in response to rucaparib treatment in vivo. Recently, the ARIEL2 Part 1 trial reported that OC with BRCA1 promoter methylation had increased levels of genomic LOH, a historical marker of HR deficiency, with some durable responses being reported [32] . To further investigate whether BRCA1 methylation sensitized HGSOC to PARPi, we focused on the four PDX harboring this epigenetic lesion. PDX models have the advantage that the human component of PDX samples is highly enriched for neoplastic cellularity in comparison with baseline patient samples. Two of the three orthogonal BRCA1 methylation assays used in this study were quantitative; either semi-quantitative (MS-HRM) or fully quantitative (MS-ddPCR), and both were human specific. As a result, we were able to observe two states of BRCA1 methylation, homozygous and heterozygous, in the four BRCA1 -methylated PDX studied. When we took into account the zygosity status of BRCA1 methylation—which importantly has not been systematically addressed in the literature with respect to clinical outcomes and association with response to PARPi or platinum [29] , [33] —we observed that the zygosity of each of the four BRCA1 -methylated PDX correlated with the zygostity status of the source tumor used to generate PDX, and did not change under the pressure of subsequent in vivo treatment of the PDX. The two chemo-naive HGSOC and corresponding PDX with homozygous BRCA1 methylation showed low BRCA1 expression by RNA-seq and responded to rucaparib in either the PDX or patient. Conversely, the two PDX with heterozygous BRCA1 methylation and some expression of BRCA1 by RNA-seq, had been generated from HGSOC treated with multiple lines of prior therapy and had failed to respond to rucaparib. In keeping with the possibility that partial loss of methylation may have occurred under treatment pressure, analysis of chemo-naive archival HGSOC samples for these two cases indicated homozygous BRCA1 methylation. These PDX studies, coupled with earlier reports correlating complete BRCA1 methylation and LOH at the BRCA1 locus [21] , provide evidence that, as is the case for BRCA1 mutated carcinomas [26] , silencing of all copies of BRCA1 by promoter methylation is required to cause an HR defect of sufficient magnitude to induce PARPi-related synthetic lethality. Consistent with these findings in PDX, we also observed that BRCA1 promoter methylation zygosity influenced PARPi response in OC cell lines. The OVCAR8 cell line has been reported to be methylated at the BRCA1 promoter, with reduction in BRCA1 mRNA and protein expression [40] , [44] , but nevertheless has been reported to be HR competent [45] . In keeping with this paradox, we found that despite having a genomic profile consistent with genomic scarring and HR deficiency [46] , OVCAR8 cells formed RAD51 foci in response to DNA damage and were resistant to PARPi in vitro, consistent with an intact HR pathway. Notably, the BRCA1 methylation status of OVCAR8 was heterozygous. In contrast, we generated a HGSOC PDX-derived cell line, WEHICS62, which retained homozygous BRCA1 methylation, had reduced ability to form RAD51 foci and was sensitive to rucaparib in vitro. The low number of cell lines reported to date with homozygous loss of BRCA1 or loss of function by mutation [40] , [47] suggests possible selection against BRCA1 -deficient cells in two-dimensional culture. Thus, the zygosity status of BRCA1 -methylated cell lines should be ascertained and re-confirmed regularly in studies where the HR status is critical. In order to investigate BRCA1 promoter methylation zygosity in clinical samples, we studied 21 high-grade OC with BRCA1 methylation from the ARIEL2 Part 1 trial [32] . Establishing the zygosity of BRCA1 methylation in patient samples was more challenging than in PDX, due to the variability in the proportion of normal stroma within each clinical sample, as well as variation in BRCA1 gene copy number. We were able to identify six high-grade OC, in which we determined with high confidence that homozygous BRCA1 methylation was present at the time of trial enrollment (in the pre-rucaparib treatment biopsy, with neoplastic cellularity >20%). Consistent with our hypothesis that homozygous methylation was required for sensitivity to rucaparib, we observed a strong association between homozygous BRCA1 methylation and rucaparib response, compared to BRCA1/2 wild-type non- BRCA1- methylated cases. It would thus be important for patient selection/stratification to use a highly quantitative method for methylation assessment, as well as accurate estimation of neoplastic cellularity and BRCA1 copy number to determine the zygosity of BRCA1 methylation, even at diagnosis, when BRCA1 -methylated cases might already have heterozygous rather than homozygous methylation. Indeed, our data strongly suggest that methylation zygosity should be assessed in contemporaneous tumor samples before any firm conclusions are drawn regarding the impact of BRCA1 methylation on therapeutic efficacy [29] , [33] . Genomic scarring assays, such as percentage genomic LOH score, are indicative of defective HR DNA repair and are likely to identify HR-defective cases with homozygous BRCA1 methylation. However, there will also be false-positive cases, where HR has been restored (e.g., through loss of methylation) yet the genomic scarring remains, reflecting a history of prior HR deficiency rather than the current HR status. In keeping with this, LOH status (percentage genomic LOH score) was not different in the BRCA1 homozygous methylated vs. “ever-methylated” cases in the ARIEL2 Part 1 trial. Furthermore, we identified cases in our clinical studies that supported the hypothesis that loss of methylation of the BRCA1 promoter could occur under platinum treatment pressure. In our PDX studies, we observed altered zygosity of BRCA1 methylation, from homozygosity in the chemo-naive archival clinical sample to heterozygosity in the previously-treated HGSOC patient source sample used to generate the PDX. Thus, heterozygous BRCA1- methylated cases may represent loss of methylation from an earlier homozygous BRCA1 methylation and HR-deficient state, contributing to PARPi resistance. A survival advantage has been demonstrated for BRCA1/2 mutated HGSOC treated with platinum-based therapies [7] , despite reversion of BRCA1/2 mutation occurring under treatment pressure [14] , [15] , [16] . However, a number of challenges may exist in demonstrating a survival advantage for BRCA1 promoter-methylated HGSOC. The first is that our data suggest that cases need to be classified according to BRCA1 methylation zygosity. The second is that homozygous BRCA1 methylation loss may occur readily under chemotherapy pressure, as our analysis of the ARIEL2 data suggests, necessitating a pre-treatment biopsy. Confirmatory studies of BRCA1 methylation zygosity in larger clinical cohorts will also be required; however, large PARPi trials in OC have focused on the maintenance setting, where tumor tissue immediately prior to PARPi has not been collected. The ARIEL2 Part 1 study is the only study to date which has routinely collected pre-treatment biopsies and which is of sufficient size to permit this analysis (204 patients enrolled with the expected case rate of BRCA1 methylation of ~10%, yielding 21 BRCA1 -methylated cases, of which 12 had homozygous methylation in the archival biopsy, eight of which had homozygous methylation in the pre-treatment biopsy (six of which were of adequate tumor purity)). Given the difficulty in accessing additional similar or larger cohorts, our data support early scheduling of PARPi treatment, for example in the first-line maintenance setting, or as combination PARPi therapy upon first relapse, to minimize the population of malignant cells in which loss of methylation and consequently resistance to treatment can occur. In summary, the study of PDX models, in which quantitative assessment of tumor BRCA1 promoter methylation is not obscured by stromal signal or complicated by variable copy number, enabled the observation that homozygous methylation and complete silencing of BRCA1 induces HR deficiency and PARPi sensitivity. By using a highly quantitative method and adjusting for neoplastic cellularity and BRCA1 copy number, we identified patients with homozygous BRCA1 methylation in the ARIEL2 Part 1 PARPi study and observed improved clinical outcomes. This study is the first to clarify the critical role of BRCA1 methylation zygosity in the response of carcinomas to PARPi and has potentially important clinical implications. Further development and refinement of methods to accurately and efficiently classify BRCA1 homozygous methylation status, and a suitably powered prospective clinical trial are required to validate our findings that homozygous BRCA1 methylation predicts PARPi sensitivity. Further, BRCA1 methylation loss in carcinomas exposed to chemotherapy underscores the importance of real-time pre-treatment biopsies to assess methylation as a predictor of response to treatment in women with recurrent HGSOC. As with secondary mutations in BRCA1/2 , loss of methylation of BRCA1 under treatment pressure disables a therapeutic mechanism of response, suggesting that earlier introduction of PARPi therapy in the disease trajectory may prevent such resistance mechanisms emerging under treatment pressure. Study approval All experiments involving animals were performed according to the animal ethics guidelines and were approved by the Walter and Eliza Hall Institute of Medical Research Animal Ethics Committee. PDX were generated from OC, with patients enrolled in the Australian Ovarian Cancer Study. Informed consent was obtained from all patients, and all experiments were performed according to the human ethics guidelines. Additional ethics approval was obtained from the Human Research Ethics Committees at the Royal Women’s Hospital and the Walter and Eliza Hall Institute. Patient samples Surgical, biopsy or ascites HGSOC samples used for PDX generation were collected from chemotherapy-naive patients who underwent surgery or patients treated with multiple lines of prior therapy. Clinical follow-up of patient outcome was obtained via the database at the Royal Women’s Hospital. Archival tumor and pre-treatment biopsy samples from 23 patients used for re-testing of BRCA1 promoter methylation were collected as part of the ARIEL2 Part 1 trial (NCT01891344) [32] . All clinical information used for interrogating rucaparib response in ARIEL2 Part 1 participating patients was collected as part of the ARIEL2 Part 1 trial [32] . Patient response was assessed according to RECIST 1.1. Generation and treatment of PDX PDX were generated as published previously by transplanting fresh fragments subcutaneously or via the intra-ovarian bursal approach into NOD/SCID/IL2Rγnull recipient mice (T1, passage 1) [34] , with the exception of PDX #169, which was generated from tumor ascites. Briefly, tumor cells were isolated from ascites after centrifugation and red blood cell lysis. The tumor cells were resuspended in diluted Matrigel Matrix (Corning) and were subcutaneously injected. Recipient mice bearing T2–T9 (passage 2 to passage 9) tumors were randomly assigned to treatment with rucaparib, cisplatin or vehicle when tumor volume reached 180–300 mm 3 . In vivo cisplatin treatments were performed as previously described [34] . The regimen for rucaparib treatment was oral gavage once daily (Monday–Friday) for 3 weeks at 150, 300, or 450 mg kg −1 . Tumors were measured twice per week and recorded in StudyLog software (StudyLog Systems). Tumors were harvested once tumor volume reached 600–700 mm 3 or when mice reached ethical endpoint. Nadir, time to progression (TTP or PD), TTH, and treatment responses are as defined previously [34] . Tumor volume and survival graphs were produced with SurvivalVolume v1.2 [48] . Median TTH was calculated by including censored events for PDX where mice were harvested when the tumor volume was >500 mm 3 but <600 mm 3 (for rucaparib response for PDX #62, 4 out of 6 mice). CR was achieved if the average tumor volume for the treatment group reduced to <50 mm 3 for two or more consecutive measurements. PR was achieved if the average tumor volume reduced to between 50 and 140 mm 3 (>30% reduction from nadir, assigned as 200 mm 3 ) for two or more consecutive measurements. SD was achieved if TTP for the treatment group was at least twice as long as TTP for the corresponding vehicle group. Cell lines and culture The human OC cell line OVCAR8 was obtained from the NCI. Early passages of the parental OVCAR8 and RAD51C KO 2–130 were cryopreserved, and were last authenticated by STR profiling in April 2017. Subsequent revivals were used within 6 months. OC cell line WEHICS62 was generated from PDX #62, by digesting cells with human tumor dissociation kit (Mitenyl Biotec) with gentleMACS dissociator, and then enriching for viable Epcam (347197 1:30; BD) positive cells using flow cytometry. Early-passage were viably stored; subsequent thaws were used within 6 months. The STR profile for WEHICS62 was generated in April 2017: Amelogenin—X; CSF1PO—allele 12; D13S317—allele 9; D16S539—allele 13; D21S11—alleles 29, 30; D5S818—allele 7; D7S820—allele 9; TH01—allele 7; TPOX—allele 8; and vWA—alleles 17, 18. The PEO4 and PEO1 cell lines were obtained from F. Couch (Mayo Clinic) in 2013 and viably stored until 2016. Subsequent thaws were used within 6 months; were last authenticated by STR profiling in April 2017. All cell lines were routinely tested and shown to be negative for Mycoplasma . Cell lines were cultured in RPMI-1640 (Corning) supplemented with 10% FBS (Peak Serum) and 1% penicillin and streptomycin (Corning) or in DMEM/F12, GlutaMAX with 5 µg ml −1 insulin, 50 ng ml −1 EGF, and 1 µg ml −1 hydrocortisone in a 5% CO 2 atmosphere at 37 °C. FT282 cells were grown in DMEM:Ham’s F12 (50:50) without HEPES in the presence of Ultroser G serum substitute. Compounds Rucaparib camsylate salt was manufactured by Lonza. Cisplatin was obtained from Pfizer. RAD51 foci formation assay For RAD51 foci assay in cell lines, cells were first treated with 10 mM EdU, then shortly after irradiated with 10 Gy. Cells were fixed 6 h post irradiation with 10% paraformaldehyde, permeabilized with 0.3% TritonX-100, blocked with blocking buffer (5% goat serum, 0.3% TritonX-100 in PBS), and incubated with rabbit anti-human RAD51 (ab63801 1:100; Abcam), followed by incubation with goat anti-rabbit 488 secondary antibody (1:600; Invitrogen). Cells were incubated for 30 min at room temperature in Click-IT reaction (100 mM Tris pH 8.5, 10 nM Alexa Fluor 647-azide (Cat# A10277, Thermo Fisher Scientific), 1 mM CuSO 4 , and 100 mM ascorbic acid), then washed with PBS. Nuclei were counterstained with DAPI in Vectashield mounting media (Vector Labs). Images were acquired on an Olympus BX-61 microscope equipped with a Spot RT camera (model 25.4), using the Spot Advanced software. EdU positive cells with more than 10 RAD51 foci/nucleus were manually scored. At least 170 cells from three independent experiments were counted. For ex vivo RAD51 foci assay, tumor tissue was first harvested, then placed in cell culturing medium and shortly after irradiated with 10 Gy or left untreated. Tissue fragments were fixed 4 h post irradiation for 2 h with 4% paraformaldehyde, then incubated in 10, 20, and 30% sucrose, embedded in Tissue-Tek® O.C.T. (optimal cutting temperature) compound (Sakura Finetek), and 4 µm sections were cut. Following antigen retrieval with pH 6 citrate buffer (Dako) in a pressure cooker, sections were permeabilized for 20 min with 0.2% Triton-X, washed in DPBS, and blocked for 30 min with blocking buffer (1% bovine serum albumin, 2% fetal bovine serum in DPBS). Sections were incubated overnight at 4 °C with rabbit anti-human RAD51 (ab133534 1:100; Abcam) or rabbit anti-human γH2AX (20E3 1:200; Cell Signaling), washed with DPBS, then incubated for 1 h at room temperature (RT) with anti-rabbit 488 secondary antibody (1:800; Invitrogen), washed with DPBS, then incubated for 1 h at RT with mouse anti-human Geminin (ab104306 1:100; Abcam), washed with DPBS, then incubated for 1 h at RT with anti-mouse 546 secondary antibody (1:800, Invitrogen) and Hoechst (1 drop ml −1 ), then washed with DPBS and mounted with Fluoromount-G® (SouthernBiotech). All antibody dilutions were done with blocking buffer. Sections were imaged using a LSM 780 inverse laser scanning microscope (Zeiss) and captured with an LSM T-PMT detector (Zeiss) using z-stacks. Z-stacks were flattened using Z projection function with maximum intensity in Fiji software. At least 230 cells from four fields of view and three independent experiments were counted. Cells with ≥5 RAD51 or γH2AX foci/geminin-positive nucleus were scored using CellProfiler (version 2.2.0, Broad Institute). Cell proliferation assay Cell count proliferation assay was performed using IncuCyte ZOOM system according to the manufacturer’s protocol. Briefly, cells were seeded (OVCAR8 at 500 cells; OVCAR8-RAD51C KO and WEHISC62 at 2000 cells) in 96-well plates and incubated overnight before adding treatments. Cells were treated for up to 14 days with rucaparib at 0.5 or 2 µM or medium. Medium with rucaparib or without rucaparib was replenished at 7 days. Colony formation assay Colony formation assay was performed on OC cell lines PEO4, PEO1, OVCAR8, and WEHICS62. Briefly, cells were seeded at 100 cells in 6-well plates and incubated overnight before adding treatments. Cells were treated with rucaparib at 5, 12.5, 25, 50, and 250 nM or equivalent amount of DMSO (no treatment control). The experiment was terminated when colonies formed in cultures without treatment (PEO4 cells fixed at 14 days; OVCAR8 and PEO1 cells fixed at 10 days; WEHICS62 cells fixed at 21 days). Colonies were fixed with 0.5% Crystal Violet and 20% methanol for 20 min. Colonies were counted blindly by three individuals, and then the average count was taken for each replicate. Immunohistochemistry Staining was performed using an automated platform with a DAKO Omnis (Agilent Pathology Solutions) on all first-generation PDX samples (T1) to confirm the retention of HGSOC characteristics when compared to the clinical pathology report, or in-house staining, at the time of sample collection. The following antibodies were used: p53 (M700101 1:100; Dako), Ki67 (M7240 1:50; Dako), Cytokeratin (M3515 1:200; Dako), PAX8 (10336–1-AP 1:20000; Proteintech), and WT1 (ab15249 1:800; Abcam). CD45 (M0701 1:500; Dako) was used to exclude donor-derived transplantable hematologic malignancy. Scoring was performed for each PDX by one investigator on one tumor section each from at least three independent mice bearing that PDX and from the relevant baseline patient tumor. Usually ten high-powered fields (for some only five were available) were surveilled and the staining estimated as follows: 3+ almost all tumor cells were strongly positive; 2+ >25% of tumor cells were strongly positive or nearly all tumor cells were moderately positive; 1+ <25% of tumor cells were moderately to strongly positive, or nearly all cells were weakly positive; 0 occasional positive cells only. Genomic analyses and qRT-PCR RNA-seq was performed on 12 baseline patient HGSOC samples used to generate PDX, and on two PDX samples (#169 and #201) to verify expression levels observed in the matched HGSOC with suboptimal sample quality due to either low neoplastic cellularity or poor RNA quality. Libraries were prepared using TruSeq RNA Library Prep Kit v2, and the sequencing was performed on the Ilumina HiSeq 2500 platform to read length of 50 bp (Australian Genome Research Facility). Reads were mapped to Human GRCh38 (GCA_000001405.15) with dbSNP150 and Ensembl 90 annotation using HISAT2 [49] , and annotated against dbSNP150 and Ensembl 90. Counts were done using HTSeq [50] , and TMM normalization was performed [51] . Expression plots were produced using Matplotlib. Baseline patient HGSOC sample #80 had to be excluded from final analysis as it failed alignment QC due to high proportion of multi-mapping reads. For qRT-PCR BRCA1 assay, RNA was converted to cDNA using Superscript III Reverse Transcriptase (Invitrogen), and qPCR was performed using SYBR Green PCR Master Mix (Applied Biosystems) following manufacturer’s instructions. 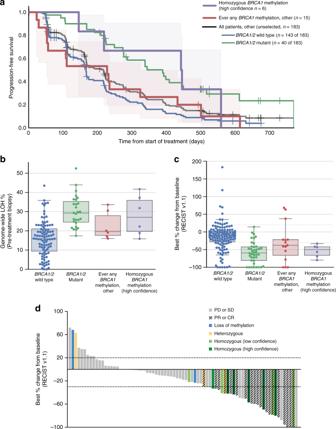Fig. 5 HomozygousBRCA1methylation and rucaparib response in the ARIEL2 Part 1 trial.aKaplan–Meier progression-free survival analysis of patients with HGSOC with homozygousBRCA1methylation in the pre-treatment tumor biopsy, which was of high confidence based on adequate neoplastic cellularity (homozygousBRCA1methylation (high confidence)), compared with patients with HGSOC in which there had ever been any other evidence ofBRCA1methylation (ever anyBRCA1methylation), compared with all other patients in the ARIEL2 Part 1 trial without anyBRCA1methylation (BRCA1/2mutant vs.BRCA1/2wild-type non-BRCA1-methylated subgroups). Shaded areas represent 95% CI for homozygousBRCA1methylation (high confidence) and ever any BRCA1 methylation, other groups.bGenome-wide LOH % assessed in the pre-treatment biopsies compared across subgroups: homozygousBRCA1methylation (high-confidence), (n= 6); ever anyBRCA1methylation, (n= 6);BRCA1/2mutant, (n= 27); andBRCA1/2wild-type non-BRCA1-methylated, (n= 96). Boxplot—median, whiskers—95% CI, dots represent individual samples.cBest percentage change from baseline in sum of longest diameter of target lesions according to RECIST 1.1 compared across subgroups: homozygousBRCA1methylation (high confidence), (n= 6); ever anyBRCA1methylation, (n= 15);BRCA1/2mutant, (n= 40); andBRCA1/2wild-type non-BRCA1-methylated, (n= 143). Boxplot—median, whiskers—95% CI, dots represent individual samples.dBest percentage change from baseline in sum of longest diameter of target lesions according to RECIST 1.1 in theBRCAwild-type LOH-high subgroup of patients byBRCA1methylation status. Each bar represents percentage change from baseline in sum of the longest diameter of target lesions for an individual patient according to RECIST 1.1. In some patients, although best percentage change of >30% was observed, the response was not investigator confirmed and thus classified as stable disease (SD) or progressive disease (PD). PR partial response, PD progressive disease, SD stable disease, CR complete response Primer sequences are listed in Supplementary Table 5 . Ct values for each sample were normalized to the average Ct values of four different housekeeping genes ( HPRT1 , ACTB , SDHA , and GAPDH ), and resulting values were used to calculate fold-change of BRCA1 expression for each sample. Baseline patient HGSOC samples used to generate PDX or PDX samples were sequenced using Foundation Medicine’s NGS-based T5a assay [52] . Analyzed data were plotted using OncoPrint. HR-DNA repair gene mutations were assessed by sequencing of PDX samples using the NGS-based BROCA assay: PDX #11, #13, #27, #29, #56, #62 were analyzed using BROCA v4 assay and were previously published [34] ; and all others were analyzed by BROCA v6 (Supplementary Data 6 ). Copy number analysis of BRCA1 was performed using MLPA-seq assay as previous described [53] . Amplicon sequencing of TP53 gene was performed on the patient HGSOC and PDX samples to estimate the neoplastic cellularity proportion. Amplicon libraries were prepared and sequenced as previously described [17] , with primers listed in the Supplementary Table 5 . Samples from the four BRCA1/2 mutant HGSOC were screened for reversion mutations by NGS and Sanger sequencing. Sanger sequencing was performed to amplify target regions in PDX #13, #19, #54, and #56. Long-range PCR was used to amplify target regions in PDX #19 and #56 samples, with primers specified in Supplementary Table 5 . Briefly, 100–120 ng of DNA was amplified with TaKaRa LA Taq polymerase (Takara Bio Inc) or Phusion Polymerase (Thermo Fisher Scientific) using the following cycling conditions: initial denaturation at 94 °C for 1 min or 98 °C for 30 s (respectively), followed by 30 cycles of 94 °C or 98 °C for 15 s, 60–62.8 °C for 30 s or 64–58 °C (−0.2 °C sec −1 ) for 20 s (respectively), and 68 °C for 15 min or 72 °C for 3 min (respectively), followed by final extension at 72 °C for 10 min. Long-range PCR products were cleaned using Agencourt AMPure XP (Beckman Coulter) beads at 1:0.4 ratio following the manufacturer’s protocol then processed using the Nextera XT DNA Library Preparation Kit (Illumina) according to manufacturer’s protocol. The libraries were sequenced using a 300-cycle MiSeq Nano Reagent Kit v2 (Illumina). Promoter methylation analysis Promoter methylation of BRCA1 PDX samples was determined by methylation-sensitive PCR as previously described [21] . BRCA1 methylation was confirmed by MS-HRM, as previously described [24] . Quantification of BRCA1 methylation levels in PDX sample series, cell lines, and ARIEL2 Part 1 patient sample series was assessed by a quantitative MS-ddPCR methodology. DNA was bisulfite converted using the EZ DNA Methylation-Lightning kit (Zymo Research). Primers were designed for a 72 bp amplicon in the BRCA1 UTR. MGB probes hybridizing to the fully methylated (VIC labeled) and the fully unmethylated sequences (FAM labeled) were used. Droplet digital PCR was performed on the Bio-Rad QX-200 system. Western blotting Nuclear lysates were prepared from snap frozen tumor fragments. Western blotting was carried out using NE-PER Nuclear and Cytoplasmic Extraction Reagents (Thermo Scientific) as previously described [54] and proteins were detected using the following antibodies: BRCA1 (OP92-MS110 1:500, Calbiochem) and Tubulin (2148 1:2000, Cell Signaling). Analysis of ARIEL2 Part 1 clinical trial cases Of 204 patients included in the ARIEL2 Part 1 clinical trial and treated with single-agent rucaparib, 23 cases had evidence of BRCA1 promoter methylation according to prior MSP analysis [32] . For these 23 cases, we assessed BRCA1 methylation in a second DNA extraction from the same tumor sample by MS-ddPCR. Two of the 23 cases were excluded from the BRCA1 -methylated subgroup because assessment did not confirm BRCA1 methylation. Of the 21 samples with BRCA1 methylation by MS-ddPCR, pre-treatment biopsies were available for 12 cases, eight of which had homozygous BRCA1 methylation, and six of these were of high confidence based on adequate neoplastic cellularity (high-confidence homozygous BRCA1 methylation, n = 6). The other 15 cases were included in the “ever any BRCA1 methylation” subgroup as they had other evidence of BRCA1 methylation, which was not high-confidence homozygous methylation in the pre-treatment biopsy. These cases were compared to all other HGSOC from the ARIEL2 Part 1 trial without any evidence of BRCA1 methylation (204 cases, minus 21 cases = 183 cases), subdivided by BRCA1/2 mutant ( n = 40 cases) and BRCA1/2 wild-type ( BRCA1/2 wild-type non- BRCA1 -methylated n = 143 cases) status. Statistics Statistical analysis was performed to compare the high-confidence homozygous BRCA1 -methylated subgroup of patients (homozygous BRCA1 methylation (high confidence), n = 6 cases) with the subgroup of cases with any other evidence of BRCA1 methylation (ever any BRCA1 methylation, n = 15 cases), or with the BRCA1/2 mutant subgroup ( n = 40) or the BRCA1/2 wild-type non- BRCA1 -methylated subgroup ( n = 143). Statistical analysis was performed in Python 3.6.1 using the pandas v0.20.2, lifelines v0.11.1, seaborn v0.8.1, matplotlib v2.0.2, and scipy v0.19.1 packages. Comparisons were made between high-confidence homozygous BRCA1 -methylated subgroup of patients and the BRCA1/2 wild-type non-methylated subgroup. No statistical comparison was made between the high-confidence homozygous BRCA1 -methylated subgroup of patients and the ever any BRCA1 methylation subgroup, as the latter group contains low confidence homozygous and ambiguous cases. Fisher Exact test was used to compare the investigator-confirmed best response, independent t -test was used to compare the minimum percentage change of target lesion, and Kaplan–Meier analysis and log rank test were used to compare PFS.